Observation of quantum-tunnelling-modulated spin texture in ultrathin topological insulator Bi2Se3films Understanding the spin-texture behaviour of boundary modes in ultrathin topological insulator films is critically essential for the design and fabrication of functional nanodevices. Here, by using spin-resolved photoemission spectroscopy with p-polarized light in topological insulator Bi 2 Se 3 thin films, we report tunnelling-dependent evolution of spin configuration in topological insulator thin films across the metal-to-insulator transition. We report a systematic binding energy- and wavevector-dependent spin polarization for the topological surface electrons in the ultrathin gapped-Dirac-cone limit. The polarization decreases significantly with enhanced tunnelling realized systematically in thin insulating films, whereas magnitude of the polarization saturates to the bulk limit faster at larger wavevectors in thicker metallic films. We present a theoretical model that captures this delicate relationship between quantum tunnelling and Fermi surface spin polarization. Our high-resolution spin-based spectroscopic results suggest that the polarization current can be tuned to zero in thin insulating films forming the basis for a future spin-switch nanodevice. A three-dimensional (3D) topological insulator (TI) is a non-trivial phase of matter that acts as an electrical insulator in the bulk but can conduct a spin-polarized current on the surface [1] , [2] , [3] , [4] , [5] , [6] , [7] , [8] , [9] , [10] , [11] , [12] , [13] , [14] , [15] , [16] , [17] , [18] , [19] . These topological surface states are characterized by a Dirac-cone-like energy–momentum dispersion relation. The novel electronic structure of TIs can be manipulated to realize various novel quantum phenomena such as spin-galvanic effects, dissipationless spin currents or neutral half-fermions for quantum information storage devices [20] , [21] , [22] , [23] , [24] , [25] . The magnitude and wavevector dependence of the spin polarization of electrons and holes are among the most important key ingredients in considerations for the design of any functional device. However, such developments have been limited because of the residual bulk conductance in currently available materials, which overwhelms the surface contribution. In addition, scattering from the extrinsic bulk states leads to the reduction of spin polarization of the surface states. One promising route to minimize bulk conductance and thus improve effective spin polarization is to work with ultrathin films where the surface-to-volume ratio is significantly enhanced [26] , [27] and surface current can potentially dominate. On the other hand, in this limit the desired spin polarization of the surface states is kinematically reduced near the metal-to-insulator transition in the ultrathin films where the spin behaviour is not known to this date [10] , [11] , [15] , [18] , [19] . To date, no systematic spin-sensitive spectroscopic experimental study has been reported in the ultrathin limit across the metal-to-insulator transition, despite the direct relevance of spins in ultrathin film limits for nanodevice fabrication as well as the potential discovery of novel topological phenomena. Studying the spin polarization in the ultrathin limit is further important to experimentally demonstrate the theoretically predicted tunable Berry’s phase in TI thin films [28] . Systematic mapping of the surface spin texture in energy, momentum space and its thickness dependence is essential to understand and interpret many transport experiments on thin film TIs that are of core interest in the current TI research. We report a systematic spin-resolved, angle-resolved photoemission spectroscopy (SR-ARPES) and spin-integrated ARPES measurements on ultrathin Bi 2 Se 3 thin films for the first time. Our measurements reveal that the spin polarization is large for larger wavevectors, and the polarization magnitude increases with reduced tunnelling, and its magnitude saturates to the bulk limit at a faster rate at large electron momenta. We observe strongly binding energy- and wavevector-dependent spin polarization for the topological surface electrons in the ultrathin gapped-Dirac-cone limit, which experimentally shows that the Dirac gap opening and the thickness-dependent topological phase transition are a result of the quantum tunnelling between the two oppositely spin-textured topological surface states. These unique spin features of ultrathin films, evidently distinct from the 3D TI, open up new possibilities for devices not possible with bulk TIs. Sample characterization Spectroscopic measurements were performed on large ultrathin Bi 2 Se 3 films prepared using the Molecular Beam Epitaxy (MBE) method on GaAs(111)A substrates ( Fig. 1a ). Each crystal layer of Bi 2 Se 3 is constituted of five atomic layer, namely Se-Bi-Se-Bi-Se, which is called quintpule layer (QL) with the thickness of ∼ 1 nm (ref. 6 ). Our MBE films grow in a self-organized quintuple layer by quintuple-layer mode, and high-quality atomically smooth films can be obtained with the desired thickness (also see Supplementary Figs 1–7 and Supplementary Notes 1–3 ). A compositional layout of the film used in our measurements is shown in Fig. 1b . To protect the surface from contamination, about 40-nm Se capping is used on the top of ultrathin Bi 2 Se 3 films. To expose the surface, the films were transferred into the ARPES chamber and heated to 250 °C at pressures lower than 1 × 10 −9 torr about an hour, which blows off the Se-capping layer. 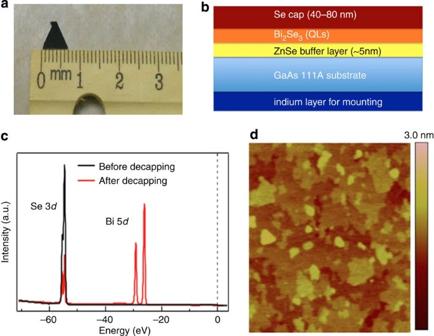Figure 1: Characterization of MBE grown ultrathin films of Bi2Se3. (a) Photograph of a representative thin film sample used in SR-ARPES measurements. (b) Sample layout of ultrathin Bi2Se3film grown by MBE. (c) Core level spectroscopy measurements on ultrathin MBE film before and after the decapping procedure. (d) Atomic force microscopy image of ultrathin Bi2Se3film. The size of the image is 1 μm × 1 μm and height is indicated by the colour bar on the right. Figure 1c shows the ARPES core level spectroscopy measurement of the ultrathin film before and after decapping of the Se layer. Before decapping, only Se peaks are visible while both Se and Bi peaks are observed after the decapping process, which proves that the Se capping works well in the ultrathin film TI system. Thin films are characterized with atomic force microscopy (see Fig. 1d ) and show that the root mean square (r.m.s.) surface roughness on these films is in the order of ∼ 0.2 nm, which confirms the high quality of the films used in our measurements. The transport measurements of the Se-capped ultrathin films result in carrier concentration, mobility and resistivity in the order of 1 × 10 19 cm −3 , 1,270 cm 2 V −1 S −1 and 0.30 mOhm cm, respectively (also see Supplementary Fig. 1 and Supplementary Note 1 ). Figure 1: Characterization of MBE grown ultrathin films of Bi 2 Se 3 . ( a ) Photograph of a representative thin film sample used in SR-ARPES measurements. ( b ) Sample layout of ultrathin Bi 2 Se 3 film grown by MBE. ( c ) Core level spectroscopy measurements on ultrathin MBE film before and after the decapping procedure. ( d ) Atomic force microscopy image of ultrathin Bi 2 Se 3 film. The size of the image is 1 μm × 1 μm and height is indicated by the colour bar on the right. Full size image Geometry of the spectroscopic measurements We used p-polarized light for our ARPES measurements. The photons approach the sample surface with angle of incident ( θ ) 45 degree with the sample normal and our samples are aligned along momentum space cut ( Fig. 2a ) for spin–ARPES measurements. The surface wavevector-dependent spin polarization is obtained using a Mott polarimeter ( Fig. 2a ), which measures two orthogonal spin components of a photoemitted electron [29] , [30] . In the polarimeter, a gold foil was used as a scattering source to generate an asymmetry of high energy photoelectrons into different divergent spin states (see refs 29 , 30 for details). Each orthogonal spin-polarization component is selected by the orientation of a scattering plane defined by the incident beam direction of the photoelectron on the gold foil and the orientation of two electron detectors mounted on each side of the foil. For this experiment, the detector configuration was set in a way that the two spin components correspond to the in-plane and out-of-plane directions of the (111) plane of the sample. 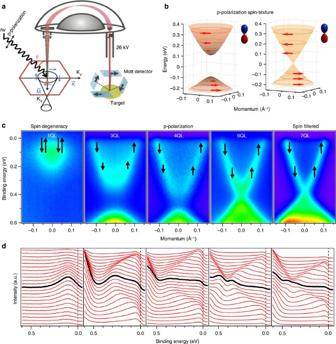Figure 2: Spin-texture versus quantum tunnelling in ultrathin Bi2Se3. (a) Experimental geometry used in our measurements. (b) Visualization of the contrasting spin configurations in 3QL (insulator) and 7QL (metal) thin films. The dumbbell signs indicate that the current experimental geometry mainly probes thepzorbitals of Bi and Se. (c) High-resolution ARPES measurements on ultrathin films of Bi2Se3:E−kband dispersion images for 1QL, 3QL, 4QL, 6QL and 7QL of Bi2Se3films taken near thepoint alonghigh-symmetry direction. The spin configuration is noted on the plots. These spectra are measured with photon energy of 60 eV. (d) The corresponding EDCs. The EDC through thepoint (solid black curve) is highlighted. Figure 2: Spin-texture versus quantum tunnelling in ultrathin Bi 2 Se 3 . ( a ) Experimental geometry used in our measurements. ( b ) Visualization of the contrasting spin configurations in 3QL (insulator) and 7QL (metal) thin films. The dumbbell signs indicate that the current experimental geometry mainly probes the p z orbitals of Bi and Se. ( c ) High-resolution ARPES measurements on ultrathin films of Bi 2 Se 3 : E − k band dispersion images for 1QL, 3QL, 4QL, 6QL and 7QL of Bi 2 Se 3 films taken near the point along high-symmetry direction. The spin configuration is noted on the plots. These spectra are measured with photon energy of 60 eV. ( d ) The corresponding EDCs. The EDC through the point (solid black curve) is highlighted. Full size image Thickness- and wavevector-dependent spin polarization We present high-resolution spin-integrated ARPES data and corresponding energy distribution curves (EDCs) along the high-symmetry line for 1QL, 3QL, 4QL, 6QL and 7QL Bi 2 Se 3 films in Fig. 2c,d . As long as the thickness of the film is comparable to the decay length of the surface states into the bulk, there is a spatial overlap between the top and bottom surface states resulting in an energy gap at the time-reversal invariant point ( point). As expected theoretically [26] , [27] , the energy gap decreases and eventually vanishes for sufficiently thick films, corresponding to the transition from a two-dimensional (2D) gapped system (insulator) to a 3D gapless system (metal) [10] , [11] . In particular, the gapless dispersion relation observed in the 7QL film from ARPES measurement indicates that this thickness is above the quantum tunnelling limit. On the basis of experimental observations, we present an illustration of the spin configuration for 3QL (insulator; see Supplementary Figs 2 and 3 and Supplementary Note 2 ) and 7QL (metal) ultrathin Bi 2 Se 3 films in Fig. 2b . It is important to note that a wide range of electronic structures have been reported in ultrathin TI films grown by MBE depending on the nature of the substrates used [10] , [11] , [18] . Different substrates result in different potential jumps from the substrate (the bottom surface of the ultrathin film) to the vacuum (the top surface of the film). When the potential is large, the Dirac point energy of the bottom surface is offset with respect to that of the top surface. Such Dirac point energy offset is observed to cause sizeable Rashba-type splitting of surface states as reported in ultrathin Bi 2 Se 3 films grown on double-layer graphene-terminated 6 H-SiC (0001) substrate [10] and Bi-terminated Si(111)-(7 × 7) (ref. 18 ) substrate by MBE, respectively. On the other hand, no observable Rashba-type splitting because of substrate potential is reported in the Bi 2 Se 3 grown on Si(111) β (3) 1/2 × (3) 1/2 -Bi substrate (in ref. 11 ), α -Al 2 O 3 (sapphire) (0001) substrate (in ref. 19 ) and our current work GaAs(111)A. We investigate the degree of spin polarization of the films as a function of electron wavevector for films of various thicknesses. To illustrate the wavevector-dependent spin polarization, 3QL film is chosen (see Supplementary Figs 2 and 3 and Supplementary Note 2 for details). The SR-ARPES data for the wavevectors, ∼ 0.05 and 0.1 Å −1 are presented in Fig. 3 . For each wavevector selected, we present a spin-resolved EDC, which shows the relative intensity of photoelectrons with up and down spin polarizations ( Fig. 3a,c ). For each such plot we associate a net spin polarization with the surface state of a given wavevector ( Fig. 3b,d ) and for 3QL film ∼ 25 and 15% are estimated at momenta ∼ 0.1 and ∼ 0.05 Å −1 , respectively. From these plots it is clearly observed that the net spin polarization decreases for smaller wavevectors (locations k ∼ 0.05 Å −1 in Fig. 3d ). The decrease can be understood as the presence of a tunnelling gap in the ultrathin limit that effectively prevents the partner-switching behaviour expected in the gapless topological surface states’ system [27] . The tunnelling gap for ultrathin films can be seen in the data ( Fig. 2c ). The reduction in the spin polarization and the existence of a tunnelling gap in the data suggest that the right-handed contribution of the bottom surface to the spin polarization must increase to effectively cancel the left-handed helical spin texture of the top surface upon approaching smaller momentum values near . 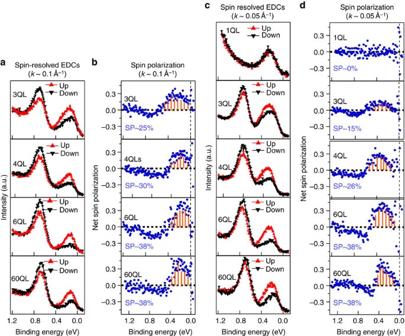Figure 3: Thickness-dependent quantum tunnelling and evolution of spin configuration. (a) Spin-resolved EDCs and (b) net tangential spin polarizations for 3QL, 4QL, 6QL and 60QL ultrathin Bi2Se3films atk∼0.1 Å−1.c,dsame asa,bfor 1QL, 3QL, 4QL, 6QL and 60QL ultrathin Bi2Se3films atk∼0.05 Å−1. The red (black) curves show tangentially up (down) spin-resolved EDCs. The magnitude of each net spin polarization is also noted in (b,d). The vertical red lines inb,dare guides to the eye, indicating a non-zero area under the spin polarization curve. SR-ARPES data were collected using photon energy of 60 eV. We note that 1 QL is equivalent to∼1 nm. Figure 3: Thickness-dependent quantum tunnelling and evolution of spin configuration. ( a ) Spin-resolved EDCs and ( b ) net tangential spin polarizations for 3QL, 4QL, 6QL and 60QL ultrathin Bi 2 Se 3 films at k ∼ 0.1 Å −1 . c , d same as a , b for 1QL, 3QL, 4QL, 6QL and 60QL ultrathin Bi 2 Se 3 films at k ∼ 0.05 Å −1 . The red (black) curves show tangentially up (down) spin-resolved EDCs. The magnitude of each net spin polarization is also noted in ( b , d ). The vertical red lines in b , d are guides to the eye, indicating a non-zero area under the spin polarization curve. SR-ARPES data were collected using photon energy of 60 eV. We note that 1 QL is equivalent to ∼ 1 nm. Full size image Figure 3a shows the spin-resolved EDCs for 3QL, 4QL, 6QL and 60QL films while the corresponding net polarization is shown in Fig. 3b at k =0.1 Å −1 . Analogous measurements are shown in Fig. 3c,d at k =0.05 Å −1 for 1QL, 3QL, 4QL, 6QL and 60QL films. For thinner films, such as 3QL, there is a naturally larger contribution from the bottom surface (because of tunnelling between top and bottom surfaces). This leads to a larger variation in spin polarization as a function of wavevector. For thicker films, this tunnelling contribution decreases and the surface spin polarization becomes more uniform with varying wavevector. For instance, in the 60QL film, no measurable change in spin polarization is observed for the variation in wavevector magnitude. Our data suggest that the magnitude of polarization tends to reach the bulk limit faster at larger wavevectors. Experimental results are summarized in Fig. 4a . Data further suggest that the relative contribution from the top surface systematically increases with film thickness. 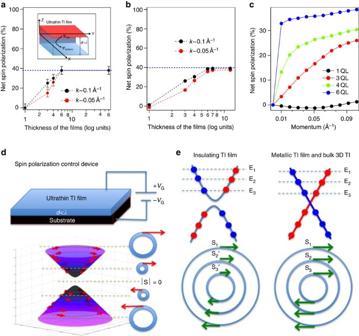Figure 4: Experimental versus theoretical spin polarization and texture. (a) Experimentally observed net spin polarization as a function of thin film thickness fork∼0.05 and 0.1 Å−1. The inset shows a schematic view of quantum tunnelling in ultrathin TI films. (b) Calculation results of spin polarization versus film thickness at two momentum pointsk∼0.05 and 0.1 Å−1. (c) Results of a calculation of the net spin polarization as a function of wavevector for ultrathin films of thickness 1QL, 3QL, 4QL and 6QL. Dashed lines ina,band solid lines incbetween the dots serve as guides to the eye. Error bars inarepresent experimental uncertainties in determining the spin polarization. Schematic of (d) a gate controlled spin polarization current switch device and (e) momentum-dependent spin configuration in ultrathin (insulating) film and thicker (metallic) film. Figure 4: Experimental versus theoretical spin polarization and texture. ( a ) Experimentally observed net spin polarization as a function of thin film thickness for k ∼ 0.05 and 0.1 Å −1 . The inset shows a schematic view of quantum tunnelling in ultrathin TI films. ( b ) Calculation results of spin polarization versus film thickness at two momentum points k ∼ 0.05 and 0.1 Å −1 . ( c ) Results of a calculation of the net spin polarization as a function of wavevector for ultrathin films of thickness 1QL, 3QL, 4QL and 6QL. Dashed lines in a , b and solid lines in c between the dots serve as guides to the eye. Error bars in a represent experimental uncertainties in determining the spin polarization. Schematic of ( d ) a gate controlled spin polarization current switch device and ( e ) momentum-dependent spin configuration in ultrathin (insulating) film and thicker (metallic) film. Full size image Model calculation First-principles theoretical modelling of the spin-polarization behaviour in thin films is presented in Fig. 4b,c . In the calculations, symmetric slabs are used to simulate the thickness of films. While a gapless spin-polarized Dirac-cone is seen on the surface of a semi-infinite crystal of the TI Bi 2 Se 3 , a gap is found to open at the Dirac point for thin films because of a finite tunnelling amplitude between the two sides of the slab surface in our calculations. The tunnelling amplitude increases as the thickness decreases, causing the gap to increase and spin polarization to decrease in the gap region. In the calculation we also consider the electron attenuation length ( ) because of the scattering processes since only electrons near the surface are able to reach the top of the surface and escape into the vacuum as in the measurement condition. Indeed, the spin polarization obtained by ARPES reflects the spin texture of the states associated with top surface rather than the bottom surface. The calculated spin expectation value for the electrons that can escape from the sample is , where d atom is the distance of an atom to the top surface, and the ‹ S › atom is the spin expectation value for each atom. The contribution from each atom is weighted by exp , which reduces the contribution from the bottom layer. Figure 4b,c shows the calculated results with , which agrees excellently with our experimental observation (see Supplementary Methods for details related to calculations). It is important to note that the maximum spin polarization observed in the bulk limit is only ∼ 40% ( Fig. 4c ), whereas the original ideal theoretical limit is that of nearly 100% without considering any specific material system [31] . In real TI materials, the strong spin–orbit interaction entangles the spin and orbital momenta of different atomic types, resulting in the reduction of spin polarization [32] . Specifically, the low-energy states in Bi 2 Se 3 arise from p -orbitals of Bi (6 p 3 ) and Se (4 p 4 ), mostly p z levels of Bi and Se [6] , [12] . The dominance of the p z orbitals in the topological surface states is further suggested by our circular dichroism measurements (see Supplementary Fig. 4 ; Supplementary Note 2 and Supplementary Methods ). The spin–orbit coupling mixes spin and orbital angular momenta while preserving the total angular momentum [6] , [12] . The hybridization of orbitals in Bi and Se together with the entanglement of their spins contribute to the reduction of net spin polarization in real materials. Moreover, under the experimental geometry used in our measurement with p-polarized light (which is most sensitive to p z orbitals and most reflective of initial ground state of the wavefunction), the penetration depth of the ARPES experiment (three to five atomic layers maximum), the experimental observation of spin polarization is well agreed with recent theoretical calculations [33] , [34] , [35] . Most importantly, our systematic spin spectroscopy results suggest that ultrathin films can serve as the basis for making qualitatively new devices, not possible with much-studied conventional 3D bulk TIs, despite the reduction of the polarization magnitude. The energy–momentum space spin texture revealed in our study provides critical knowledge to design and interpret devices based on ultrathin films. For spintronics applications, our results suggest that ultrathin TI films can be used to fabricate new types of nanodevices because of the novel spin configurations and their systematic modulations possible in the ultrathin limit. One such potential application implied by our spectroscopic results is that of a polarization current switch. Spin spectroscopic results suggest that it should be possible to control the polarization magnitude by varying a gate voltage ( Fig. 4d,e ) across a high-quality insulating thin film (see supplementary Fig. 5 and Supplementary Note 3 ). Such electrostatic gating would be similar to the in situ chemical gating by K-deposition and NO 2 adsorption shown in Supplementary Figs 6 and 7 , where the surface state structure does not change appreciably, while the Fermi energy is moved from regions of high polarization to low polarization (see Supplementary Note 3 ). This effect, which cannot be readily realized in the highly polarized states of conventional 3D bulk TIs, allows ultrathin TI films to serve as the basis for functional nanodevices, which can encode electrical signals in varying spin polarization magnitude or forms the physical basis for a spin switch, among many other new application possibilities suggested by our observations of the fundamental spin modulation behaviour in ultrathin films. Sample growth and transport measurements Ultrathin Bi 2 Se 3 films used for this study were synthesized by MBE on a GaAs(111)A substrate with a ZnSe buffer layer. Details of sample preparation are described elsewhere [36] , [37] . To protect the surface from oxidation, a thick Se-capping layer was deposited on the Bi 2 Se 3 thin film immediately after growth. To achieve the clean Bi 2 Se 3 surface required for photoemission measurements, thin films were heated up inside the ARPES chamber to 250 °C under vacuum better than 1 × 10 −9 torr to remove the Se-capping layer on top of ultrathin Bi 2 Se 3 . Hall bars fabricated from the Se-capped samples had carrier concentrations in the 1–2 × 10 19 cm −3 range. Transport measurements were carried out on Hall bars of the 5 and 6QL thick films with the Se-capping layer in place by standard photolithography and dry etching and were measured at 4.2 K. High-resolution ARPES measurements High-resolution spin-integrated ARPES measurements were performed with 29–64 eV photon energy on beamlines 10.0.1 and 12.0.1 at the Advanced Light Source in Lawrence Berkeley National Laboratory. Both endstations were equipped with a Scienta hemispherical electron analyser (see VG Scienta manufacturer website ( http://www.vgscienta.com/ ) for instrument specifications). The typical energy and momentum resolutions were 15 meV and 1% of the surface Brillouin zone, respectively, for spin-integrated measurements. Spin-resolved ARPES measurements Spin-resolved ARPES measurements were performed at the UE112-PGM1 beamline at Bessy II in Berlin, Germany, and the I3 beamline at Maxlab in Lund, Sweden, using classical Mott detectors and photon energies 55–60 and 8–20 eV, respectively. The typical energy and momentum resolutions were 100 meV and 3% of the surface Brillouin zone for spin-resolved measurements. All the SR spectra presented are measured in BESSY II unless it is specified. Theoretical calculations The first-principles calculations for spin polarizations of ultrathin films are based on the generalized gradient approximation [38] using the full-potential projected augmented wave method [39] , [40] as implemented in the VASP package [41] . The 1QL, 3QL, 4QL, 6QL, 7QL and 12QL slab models with a vacuum thickness larger than 10 Å are used in this work. The electronic structure calculations were performed over 11 × 11 × 1 Monkhorst-Pack k-mesh with the spin–orbit coupling included self-consistently. How to cite this article: Neupane, M. et al. Observation of quantum-tunnelling-modulated spin texture in ultrathin topological insulator Bi 2 Se 3 films. Nat. Commun. 5:3841 doi: 10.1038/ncomms4841 (2014).